[3+2] Cycloaddition of alkyl aldehydes and alkynes enabled by photoinduced hydrogen atom transfer [3+2] Cycloaddition is a step- and atom-economic method for the synthesis of five-membered rings. Despite the great success of 1,3-dipolar cycloadditions, the radical [3+2] annulation of alkynes remains a formidable challenge. Herein, a photoinduced decatungstate-catalyzed [3+2] cycloaddition of various internal alkynes using abundant aliphatic aldehydes as a three-carbon synthon is developed, producing elaborate cyclopentanones in 100% atom economy with excellent site-, regio-, and diastereoselectivity under mild conditions. The catalytic cycle consists of hydrogen atom abstraction from aldehydes, radical addition, 1,5-hydrogen atom transfer, anti-Baldwin 5-endo-trig cyclization, and back hydrogen abstraction. The power of this method is showcased by the late-stage elaboration of medicinally relevant molecules and total or formal synthesis of (±)-β-cuparenone, (±)-laurokamurene B, and (±)-cuparene. Cyclopentanones are important structural scaffolds embedded in a number of natural products, pharmaceuticals, and bioactive compounds, such as PGE 2 , loxoprofen, and deconin B (Fig. 1a ) [1] , [2] , [3] . Meanwhile, they can serve as versatile intermediates in synthetic chemistry. Consequently, enormous efforts have been devoted to the construction of these motifs, including the ring expansion [4] , [5] , [6] , carbene insertion [7] , [8] , and intramolecular hydroacylation [9] , [10] . However, the aforementioned methods rely on the use of prefunctionalized substrates that require multistep synthesis, thus calling for the development of more straightforward and robust protocols. Fig. 1: Background and summary of this work. 3C three carbon. TIPS triisopropylsilyl. EWG electron-withdrawing group. W tetra- n -butylammonium decatungstate. a Representative bioactive molecules bearing cyclopentanones. b Traditional [3+2] cycloaddition reactions. c This work, a radical [3+2] cycloaddition enabled by multiple HAT. Full size image The [3+2] cycloaddition represents a powerful means for assembling five-membered hetero- and carbocycles from readily attained starting materials (Fig. 1b ). In this respect, the preparation of cyclopentanones has been rarely accomplished [11] , [12] , [13] , [14] , [15] , [16] , [17] , [18] , [19] , mainly due to the lack of suitable three-carbon (3C) synthons. By harnessing the in situ generated oxyallyl cations as a 1,3-dipole, Kuwajima reported a rapid assembly of cyclopentanones via the [3+2] cycloaddition of electron-rich and -neutral alkenes [11] . Using palladium-oxyallyl species as a 3C source, annulations of the more challenging nitroalkenes [12] , 1,3-dienes [13] , and acrylonitriles [14] were successfully developed by the groups of Zi and Wu. Kerrigan and co-workers discovered a dual Lewis acid-catalyzed [3+2] carbocyclization of ketenes with donor-acceptor cyclopropanes [15] . Alternatively, Rovis disclosed that enals could serve as a 3C building block for the access to cyclopentanones via the N -heterocyclic carbene-catalyzed cascade cyclizations [16] , [17] . Despite these significant advances, it is still highly desirable to develop novel [3+2] annulation for the atom-economic and controllable synthesis of polysubstituted cyclopentanones, particularly using readily available 3C synthons. In light of recent developments on decatungstate-catalyzed C-H functionalization of aldehydes [20] , [21] , [22] , [23] , [24] , [25] , [26] , [27] , [28] , [29] , [30] , [31] , [32] , [33] and our interest [34] on 5-endo-trig radical cyclization of all-carbon systems, we envisioned that abundant aliphatic aldehydes could be exploited as an ideal 3C component for the [3+2] carbocyclization of alkynes via the hydrogen atom transfer (HAT) [35] , [36] , [37] , [38] , [39] , [40] -induced double C-H functionalization (Fig. 1c ). In this work, we report a photoinduced tetra- n -butylammonium decatungstate (TBADT) catalyzed radical [3+2] cycloaddition of alkyl aldehydes and a wide range of alkynes, which provides a streamline and robust access to heavily functionalized cyclopentanones from readily attained feedstocks. In contrast to the traditional ionic protocols [11] , [12] , [13] , [14] , [15] , [16] , [17] , [18] , this single-electron-mediated process exhibits many advantages, such as mild and redox-neutral conditions, 100% atom economy, excellent site-, regio-, and diastereoselectivity, very broad substrate scope, and high efficiency, rendering it an attractive strategy for chemical synthesis and drug discovery. Reaction optimization Optimization studies began with the reaction of commercially available alkyl aldehyde 1a and alkyne 2a . 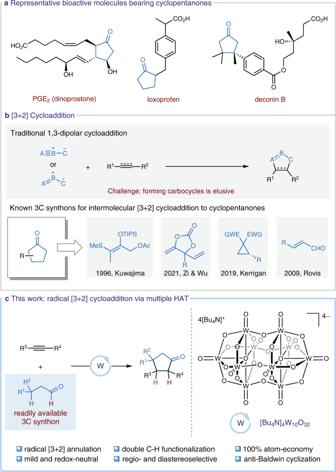Fig. 1: Background and summary of this work. 3C three carbon. TIPS triisopropylsilyl. EWG electron-withdrawing group. W tetra-n-butylammonium decatungstate.aRepresentative bioactive molecules bearing cyclopentanones.bTraditional [3+2] cycloaddition reactions.cThis work, a radical [3+2] cycloaddition enabled by multiple HAT. Upon treating the reaction mixture with 2 mol% of TBADT under irradiation of 40W, 390 nm purple LEDs in a 10:1 mixture of MeCN and H 2 O at 25 °C for 10 h, cyclopentanone 3 was isolated in 88% yield as a single regio- and diastereoisomer (Table 1 , entry 1). Switching the HAT photocatalyst from TBADT to NaDT resulted in a slightly decreased yield (entry 2). Other reaction mediums, such as MeCN, DMSO, acetone, and DMF, proved to be less effective (entries 3–6). The controlled experiments revealed that both TBADT and light are essential for this transformation (entries 7 and 8). Table 1 Optimization of reaction conditions Full size table Examination of substrate scope Having established the optimized reaction conditions, we set about investigating the scope of this [3+2] annulation with various functionalized alkynes (Fig. 2 ). Arylalkynyl esters were first evaluated. Pleasingly, they worked well for this reaction and produced a set of decorated cyclopentanones, including those possessing fluorine, chlorine, or bromine atom on the benzene ring, in high yields with excellent regio- and diastereoselectivity ( 4 - 8 ). The trans -diastereoselectivity was confirmed by the single X-ray diffraction analysis of 6 . In contrast, the reaction of alkylalkynyl esters formed the kinetically favorable cis -2,3-disubstituted cyclopentanones 9 and 10 in high yields, whose structures were assigned by NMR measurements (see the Supporting Information for details). Polar effect, instead of the radical delocalization to the neighboring aryl group that dominates in the transformation of arylalkynes, may account for the reversed regioselectivity [41] . Of note, trans -2,3-disubstituted cyclopentanones 11 and 12 could be selectively obtained in satisfactory yields via a subsequent NaOH-promoted epimerization, further enhancing the utility of this method. Fig. 2: Scope of the reaction. Reaction conditions: see Table 1 , entry 1; Isolated yields are given. Unless otherwise noted, the desired products were obtained with ≥10:1 dr selectivity. b Yield of 1.0 mmol scale. c (i) see Table 1 , entry 1; (ii) NaOH (0.2 mmol), EtOH, RT, 5 h. d (i) see Table 1 , entry 1; (ii) K 2 CO 3 (0.4 mmol), DMSO, 80 °C, 5 h. Dr diastereoisomer ratio. TBS tert -butyldimethylsilyl. RT room temperature. Full size image Given the versatile reactivity of carbon-halide bonds, we then tested the reactivity of alkynyl chlorides. To our delight, they served as efficient substrates to form various trans -2,3-disubstituted cyclopentanones in promising yields with high regio- and diastereoselectivity. A large number of functional groups, such as fluorine ( 14 ), chlorine ( 15 and 22 ), bromine ( 16 ), methoxyl ( 19 , 26 , and 27 ), ester ( 20 ), nitrile ( 21 ), and terminal alkyne ( 25 ) were well tolerated, leaving ample room for further functionalizations. The single X-ray diffraction crystallography identified the structure of 13 . This process was well amenable to chloroalkynes bearing heterocycles, such as pyridine and thiophene, which delivered cyclopentanones 28 - 30 in 68–87% yields, without erosion of the site-, regio-, and diastereoselectivity. In addition to arylalkynyl chlorides, we also evaluated the reaction of alkenyl counterpartners, a class of challenging substrates due to the potential radical addition to C-C double bonds. As an example, cyclohexenyl ethynylchloride produced the alkenyl cyclopentanone 31 in 75% yield, highlighting the high chemoselectivity of this reaction. Remarkably, the double [3+2] cycloaddition was quite successful, as demonstrated by the regio- and diastereoselective construction of 32 and 33 , in which eight new chemical bonds and two carbocycles were concurrently assembled. As demonstrated by the production of 34 , alkylalkynyl chlorides also served as the competent coupling partner, albeit with a decreased diastereoselectivity (dr = 5:1). Meanwhile, we examined the reaction of phenylethynyl bromide, however, it failed to provide the annulation product due to the formation of alkynyl ketone 36 via a radical addition/β-elimination sequence. On the other hand, alkynyl nitrile proved to be a viable substrate, exclusively forming the trans -2,3-disubstituted cyclopentanone 38 in nearly quantitative yield. The carbocyclization of 1-phenyl-1-propyne, a weakly activated alkyne, took place efficiently to furnish 39 in 89% yield, however, a low diastereoselectivity (dr = 1.9:1) was observed. After some trials, the dr value could be improved to >20:1 upon combining with a subsequent K 2 CO 3 -promoted epimerization, implying that the trans -diastereoselectivity is thermodynamically controlled. In contrast, terminal alkynes were sluggish for this annulation ( 41 ). The applicability of this reaction with respect to aldehydes was briefly examined. A set of aliphatic aldehydes with tertiary C-H bonds reacted uneventfully to afford the synthetically important but challenging spirocyclopentanones 42 - 44 in 73–93% yields with high diastereoselectivity. Cyclopentanone 45 , bearing three continuous stereocenters, was selectively constructed under the reaction conditions. Substitution of the aldehyde with OTBS and OH groups had no detrimental effect on this cycloaddition, delivering elaborate cyclopentanones 46 and 47 in satisfactory yields. In contrast, 2-cyclohexylpropanal ( 1h ) and aldehydes with a set of secondary C-H bonds ( 1i - 1m ) were almost unreactive under the identical conditions. Then, we performed the late-stage modifications of drug-related compounds via this protocol. In particular, estrone, an estrogenic hormone, was converted into cyclopentanone 48 in 80% yield; clofibrate and fenofibrate, two cardiovascular drugs, were transformed to 49 and 50 in 91% and 87% yield, respectively; celecoxib, an anti-inflammatory agent, provided cyclopentanone 51 in high yield. Synthetic applications To illustrate the synthetic utility of this radical [3+2] process, 2-chlorocyclopentanone 17 was treated with K 2 CO 3 in DMF at 80 °C (Fig. 3 ). As a result, cyclopentenone 52 was generated via HCl elimination in excellent yield. 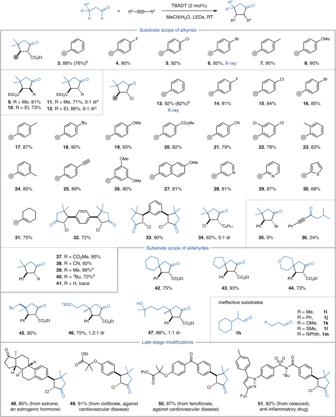Fig. 2: Scope of the reaction. Reaction conditions: see Table1, entry 1; Isolated yields are given. Unless otherwise noted, the desired products were obtained with ≥10:1 dr selectivity.bYield of 1.0 mmol scale.c(i) see Table1, entry 1; (ii) NaOH (0.2 mmol), EtOH, RT, 5 h.d(i) see Table1, entry 1; (ii) K2CO3(0.4 mmol), DMSO, 80 °C, 5 h. Dr diastereoisomer ratio. TBStert-butyldimethylsilyl. RT room temperature. A subsequent methylation using LiHMDS and MeI delivered 53 in 84% yield. Since its transformation to the antifungal and cytotoxic natural product laurokamurene B ( 54 ) [41] has been documented before, the formal synthesis of (±)- 54 [42] , [43] , [44] , [45] was thus achieved. Additionally, Ni-catalyzed conjugate addition of AlMe 3 to 52 provided 83% yield of β-cuprenone ( 55 ) [46] , [47] , [48] , [49] , [50] , a cyclopentanoid sesquiterpene used for the treatment of fungal infection, coughs, cancer, and hemorrhages. The total synthesis developed here requires only two steps from 17 and produces 55 in 77% overall yield, which compares favorably with the previous reports on the synthesis of (±)- 55 [47] , [48] . Another small-molecule natural product, cuparene ( 56 ), can also be accessible via the Wolff-Kishner reduction of 55 [49] . Fig. 3: Synthetic applications. Reaction conditions: a 17 , K 2 CO 3 , DMF, 80 °C; b 52 , LiHMDS, MeI, THF, −78 °C to RT; c 52 , Ni(acac) 2 , AlMe 3 , THF, RT. LiHMDS lithium bis(trimethylsilyl)amide. Full size image Mechanistic investigations To confirm the in-situ formation of acyl radicals, the model reaction was conducted in the presence of 2.0 equiv of TEMPO (Fig. 4 ). As a result, the TEMPO-adduct 57 , instead of cyclopentanone 42 , was isolated in 38% yield. Some deuterium-labeling experiments were then conducted. Almost no deuterium incorporation was observed with CD 3 CN as the solvent, while [D]- 42 was formed with 72% deuterium incorporation by running the reaction in a mixture of MeCN and D 2 O. In contrast, the [3+2] annulation between [D]- 1b (98% D) and 2a in MeCN produced [D]- 42 with 60% deuterium incorporation, supporting that the hydrogen atom at the C2 position of cyclopentanones comes from aldehydes. 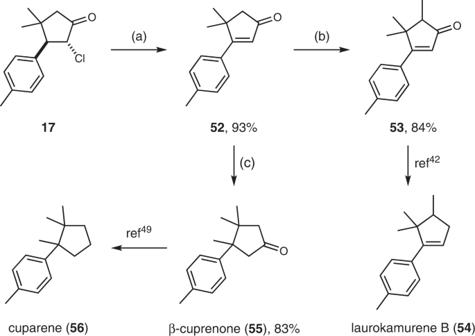Fig. 3: Synthetic applications. Reaction conditions:a17, K2CO3, DMF, 80 °C;b52, LiHMDS, MeI, THF, −78 °C to RT;c52, Ni(acac)2, AlMe3, THF, RT. LiHMDS lithium bis(trimethylsilyl)amide. Subjection of [D]- 1b’ (75% D) to the identical conditions resulted in the generation of [D]- 42' (73% D), which is consistent with an intramolecular 1,5-HAT. Fig. 4: Mechanistic studies. TEMPO 2,2,6,6-tetramethylpiperidinooxy. Full size image Based on the above results and previous reports [20] , [21] , [22] , [23] , [24] , [25] , [26] , [27] , [28] , [29] , [30] , [31] , [32] , [33] , a plausible mechanism for this TBADT-catalyzed [3+2] cycloaddition is proposed in Fig. 5 . Initially, the excited-state catalyst *[W 10 O 32 ] 4− , obtained by photoexcitation of the decatungstate anion at 390 nm, abstracts a hydrogen atom from aldehydes to form acyl radicals I and [W 10 O 32 ] 5− H + . Subsequent radical addition to alkynes followed by 1,5-HAT of vinyl radicals [51] , [52] , [53] , [54] , [55] , [56] , [57] , [58] , [59] , [60] , [61] , [62] , [63] , [64] , [65] , [66] , [67] , [68] generates nucleophilic alkyl radicals III . Then, a polarity-matched addition at the β-carbon atom leads to radicals IV . Of course, spin delocalization to the adjacent carbonyl group may also facilitate the uncommon 5-endo-trig cyclization. Back hydrogen abstraction from the reduced form of the tungstate anion [W 10 O [32] ] 5- H + produces 3 – 51 , accompanied by restoring the TBADT catalyst. Fig. 5: Proposed mechanism. HA hydrogen abstraction. Full size image We have developed a radical [3+2] annulation of alkynes using readily accessible alkyl aldehydes as a 3C building block and TBADT as a photocatalyst. The reaction occurs under mild, redox-neutral conditions, producing a diverse array of polysubstituted cyclopentanones in 100% atom economy with high efficiency and excellent site-, regio-, and diastereoselectivity. Preliminary studies indicate a mechanism involving an intermolecular HAT, radical addition, 1,5-HAT, unusual 5-endo-trig cyclization, and back hydrogen atom abstraction. The synthetic utility of this protocol is well illustrated by the late-stage derivatizations of drug-relevant compounds, total synthesis of (±)-β-cuprenone, and formal syntheses of (±)-laurokamurene B and (±)-cuparene, thus providing an appealing method for the fast construction of biologically active molecules and natural products. 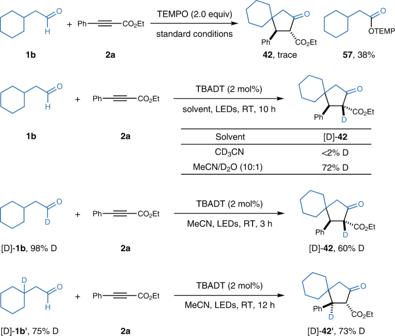Fig. 4: Mechanistic studies. TEMPO 2,2,6,6-tetramethylpiperidinooxy. 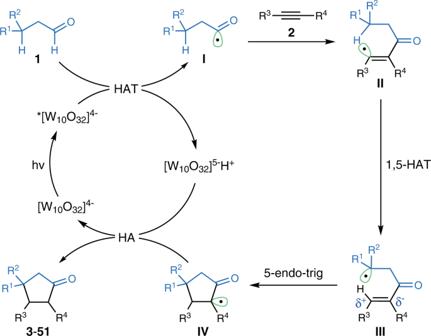Fig. 5: Proposed mechanism. HA hydrogen abstraction. Procedure for the TBADT-catalyzed [3+2] cycloaddition of alkyl aldehydes and alkynes To a mixture of TBADT (10.6 mg, 0.004 mmol) in 2 mL of MeCN/H 2 O (v:v = 10:1) was added 1a (34.4 mg, 0.4 mmol) and 2a (34.8 mg, 0.2 mmol) under nitrogen atmosphere. After 10 h of irradiation with purple LEDs (100% intensity, Kessil PR160, 40 W, 390 nm, light irradiance at a distance of 3 cm: 76.41 mW/cm [2] , and the light irradiance at the reaction site: 4.62 mW/cm [2] ), the reaction mixture was quenched with water, extracted with EtOAc, washed with brine, dried over anhydrous Na 2 SO 4 , and concentrated. The resulting residue was purified via column chromatography on silica gel to afford the desired product.